Endocannabinoid-Goα signalling inhibits axon regeneration inCaenorhabditis elegansby antagonizing Gqα-PKC-JNK signalling The ability of neurons to regenerate their axons after injury is determined by a balance between cellular pathways that promote and those that inhibit regeneration. In Caenorhabditis elegans , axon regeneration is positively regulated by the c-Jun N-terminal kinase mitogen activated protein kinase pathway, which is activated by growth factor-receptor tyrosine kinase signalling. Here we show that fatty acid amide hydrolase-1, an enzyme involved in the degradation of the endocannabinoid anandamide (arachidonoyl ethanolamide), regulates the axon regeneration response of γ-aminobutyric acid neurons after laser axotomy. Exogenous arachidonoyl ethanolamide inhibits axon regeneration via the Goα subunit GOA-1, which antagonizes the Gqα subunit EGL-30. We further demonstrate that protein kinase C functions downstream of Gqα and activates the MLK-1-MEK-1-KGB-1 c-Jun N-terminal kinase pathway by phosphorylating MLK-1. Our results show that arachidonoyl ethanolamide induction of a G protein signal transduction pathway has a role in the inhibition of post-development axon regeneration. An axon's ability to regenerate after damage is influenced by a balance of extrinsic factors that inhibit or promote axon outgrowth, as well as by intrinsic processes that regulate axon growth potential [1] . In adult mammals, the peripheral nervous system is able to regenerate, whereas the regenerative capacity of neurons in the central nervous system (CNS) is limited. This distinction between central and peripheral axon regeneration reflects differences both in intrinsic growth capacities and in the local extracellular environment [1] . For example, signalling by some myelin-associated factors such as Nogo has been suggested to be part of the reason why neurons in the CNS almost never regenerate [2] . However, recent results suggest that additional signals exist that downregulate the regenerative capacity of CNS neurons [3] . Understanding these regeneration-inhibiting pathways could have significant clinical impact and warrant further study. The nematode Caenorhabditis elegans has recently emerged as a tractable model for studying regenerative processes in neurons [4] , [5] . In particular, the amenability of C. elegans to genetic analysis should facilitate the discovery of novel molecular pathways that regulate neuronal regeneration. Recent genetic studies have shown that C. elegans axon regeneration is regulated by the p38 and c-Jun N-terminal kinase (JNK) mitogen activated protein kinase (MAPK) pathways, which consist of DLK-1 (MAPKKK)-MKK-4 (MAPKK)-PMK-3 (MAPK) and MLK-1(MAPKKK)-MEK-1(MAPKK)-KGB-1 (MAPK), respectively [5] , [6] , [7] . These MAPK cascades can be inactivated by the MAPK phosphatase VHP-1 (7,8). Indeed, axon regeneration is enhanced in a vhp-1 loss-of-function mutant because of hyperactivation of the MAPK pathways [7] . In a previous effort to identify additional components involved in MAPK-mediated signalling, we isolated 10 genes that function as suppressors of vhp-1 , which we designated svh ( s uppressor of vh p-1 ) [9] . Two of these, svh-1 and svh-2 , encode a growth factor and its cognate receptor tyrosine kinase, respectively. This SVH-1-SVH-2 signalling cascade regulates axon regeneration via the KGB-1 JNK pathway [9] ( Fig. 1a ). The involvement of the JNK pathway in axon regeneration has also been shown in vertebrates [10] , [11] . Moreover, inhibition of JNK signalling has no apparent effect on axon outgrowth during development, but dramatically affects regenerating neurites in the adult [12] . 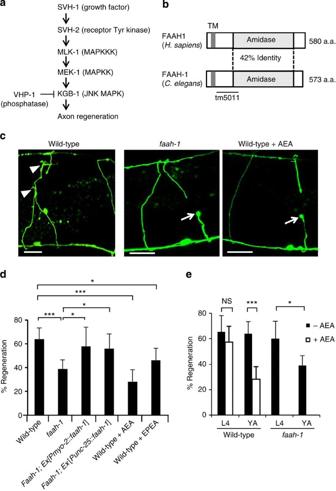Figure 1: Effects of FAAH-1 and AEA on axon regeneration inC. elegans. (a) Schematic diagram of the JNK MAPK pathway involved in axon regeneration inC. elegans. SVH-1 growth factor and SVH-2 receptor tyrosine kinase positively regulate the JNK pathway. VHP-1 MAPK phosphatase negatively regulates it. (b) Structure of FAAH-1. Comparison betweenC. elegansFAAH-1 and human FAAH1 is shown. TM represents the putative transmembrane domain. The bold line underneath indicates the extent of the deleted region in thefaah-1(tm5011)mutation. (c) Representative D-type motor neurons in wild-type andfaah-1mutant animals 24 h after laser surgery. Young adult animals were treated with ethanol or AEA for 6 h after axotomy. In wild-type animals, severed axons have regenerated growth cones (arrowheads). Infaah-1mutants and AEA-treated wild-type animals, severed axons failed to regenerate (arrows). Scale bars=10 μm. (d) Percentages of axons that had initiated regeneration 24 h after laser surgery. Young adult animals were treated with ethanol, AEA or EPEA for 6 h after axotomy. At least 30 axons per treatment group were assayed. (e) Effect of age on axon regeneration. Animals in L4 or young adult (YA) stage were treated with ethanol (−AEA) or AEA for 6 h after axotomy. Error bars indicate 95% confidence intervals (CI). *P<0.05, ***P<0.001 as determined by Fisher's exact test. NS, not significant. Figure 1: Effects of FAAH-1 and AEA on axon regeneration in C. elegans . ( a ) Schematic diagram of the JNK MAPK pathway involved in axon regeneration in C. elegans . SVH-1 growth factor and SVH-2 receptor tyrosine kinase positively regulate the JNK pathway. VHP-1 MAPK phosphatase negatively regulates it. ( b ) Structure of FAAH-1. Comparison between C. elegans FAAH-1 and human FAAH1 is shown. TM represents the putative transmembrane domain. The bold line underneath indicates the extent of the deleted region in the faah-1(tm5011) mutation. ( c ) Representative D-type motor neurons in wild-type and faah-1 mutant animals 24 h after laser surgery. Young adult animals were treated with ethanol or AEA for 6 h after axotomy. In wild-type animals, severed axons have regenerated growth cones (arrowheads). In faah-1 mutants and AEA-treated wild-type animals, severed axons failed to regenerate (arrows). Scale bars=10 μm. ( d ) Percentages of axons that had initiated regeneration 24 h after laser surgery. Young adult animals were treated with ethanol, AEA or EPEA for 6 h after axotomy. At least 30 axons per treatment group were assayed. ( e ) Effect of age on axon regeneration. Animals in L4 or young adult (YA) stage were treated with ethanol (−AEA) or AEA for 6 h after axotomy. Error bars indicate 95% confidence intervals (CI). * P <0.05, *** P <0.001 as determined by Fisher's exact test. NS, not significant. Full size image In the present study, we investigate the role of another svh gene, svh-3 , in the regulation of axon regeneration. The svh-3 gene encodes an enzyme involved in the degradation of anandamide, a well-conserved member of the endocannabinoid group. The endocannabinoid system is a lipid signalling system that regulates diverse processes such as motor control, cognition and emotional responses and is conserved in a wide variety of organisms from worms to vertebrates [13] , [14] . Anandamide was the endocannabinoid first described, and is a major ligand in this system [14] . Although some studies identify anandamide as a regulator of axonal guidance [15] , no involvement of anandamide in axon regeneration has been reported. Here, we identify anandamide signalling as an inhibitor of axon regeneration in mature C. elegans neurons. The svh-3 gene is a homologue of fatty acid amide hydrolase In order to find additional regulators of the p38 and JNK MAPK pathways in C. elegans , we performed a genome-wide RNA interference (RNAi) screen for suppressors of vhp-1 lethality [9] . Two of these svh genes, svh-1 and svh-2 , indeed regulate axon regeneration via the KGB-1 JNK pathway, as was recently demonstrated [9] ( Fig. 1a ). Another of the svh genes identified in our screen was svh-3 , which encodes fatty acid amide hydrolase-1 (FAAH-1; 13), a C. elegans homologue of the mammalian f atty a cid a mide h ydrolase FAAH ( Fig. 1b ; Supplementary Fig. S1 ). We examined the physiological function of svh-3 / faah-1 by a reverse genetic approach using the deletion mutation tm5011 , which is a loss-of-function mutant of the faah-1 gene ( Fig. 1b ). The tm5011 deletion allele is null ( Supplementary Fig. S2 ) and showed no obviously altered phenotype with respect to growth, movement or egg laying (data not shown). Anandamide inhibits axon regeneration To test whether FAAH-1 functions in axon regeneration, we assayed regrowth after laser axotomy in γ-aminobutyric acid (GABA)-releasing D-type motor neurons, which extend their axons from the ventral to the dorsal nerve cord [4] , [5] ( Fig. 1c ). In young adult wild-type animals, laser-severed axons were able to initiate regeneration within 24 h ( Fig. 1c,d ; Supplementary Table S1 ). By contrast, the frequency of axon regeneration in faah-1(tm5011) mutants was reduced ( Fig. 1c,d ; Supplementary Table S1 ) and did not recover even 3 days after surgery ( Supplementary Table S1 ). However, the morphology of D-type motor neurons was normal in faah-1 mutants (data not shown). Thus, FAAH-1 is not required for the normal development of neurons, but is required for efficient axon regeneration after laser surgery. We next examined the expression pattern of the faah-1 gene. We constructed a transgene consisting of the faah-1 promoter driving the fluorescent protein GFP that is, green fluorescent protein, Pfaah-1::gfp . As observed previously [13] , expression of Pfaah-1::gfp was detected in the pharynx and the posterior intestine ( Supplementary Fig. S3 ). We found that expression of faah-1 complementary DNA (cDNA) either by the pharyngeal muscle-specific myo-2 promoter or by the D-type motor neuron-specific unc-25 promoter was able to rescue the faah-1 defect ( Fig. 1d ) ( Supplementary Table S1 ). Thus, FAAH-1 appears to function at least in the pharynx, and possibly in the D-type motor neurons as well. FAAH is an enzyme involved in endocannabinoid degradation [16] . The endocannabinoid system regulates numerous neuronal processes such as pain perception in the hindbrain and memory-modulating synaptic plasticity in the hippocampus [14] . As RNAi knockdown of faah-1 levels results in increased levels of endogenous anandamide (arachidonoyl ethanolamide, AEA) and eicosapentaenoyl ethanolamide (EPEA) in C. elegans [13] , we hypothesised that exogenous AEA or EPEA might inhibit axon regeneration. We found that the frequency of axon regeneration of D-type motor neurons in young adult wild-type animals was reduced in the presence of AEA ( Fig. 1d ; Supplementary Table S1 ). Addition of AEA had no effect on the morphology of the neurons (data not shown). Compared with AEA treatment, EPEA had a weaker effect on axon regeneration ( Fig. 1d ; Supplementary Table S1 ). These results suggest that high levels of AEA inhibit axon regeneration after laser surgery. Interestingly, we found that animals at the fourth larval (L4) stage were insensitive to the effects of exogenous AEA on regeneration ( Fig. 1e ; Supplementary Table S1 ). Similarly, axon regeneration in faah-1(tm5011) mutants was reduced only in young adult animals, but not in L4 larvae ( Fig. 1e ). Thus, AEA inhibits regeneration after laser surgery specifically in the adult stage. AEA inhibits Gqα-PKC pathway via Goα in axon regeneration We next tried to identify the downstream signalling components that mediate the effect of AEA on axon regeneration. Endocannabinoids activate G protein-coupled cannabinoid receptors in mammals [17] , [18] but the homologous receptors in C. elegans have yet to be identified [19] . By contrast, the G proteins have distinct worm homologues. We therefore examined whether a heterotrimeric guanine nucleotide-binding protein may mediate the inhibitory effect of AEA on axon regeneration. The goa-1 gene encodes the orthologue of mammalian Goα [20] , [21] . In the loss-of-function goa-1(n1134) mutant, axons were observed to regenerate normally after laser axotomy, even in the presence of AEA ( Fig. 2a ; Supplementary Table S1 ). This indicates that the loss-of-function goa-1 mutation causes insensitivity to AEA and raises the possibility that AEA activates GOA-1, leading to inhibition of axon regeneration. Consistent with this possibility, we found that expression of a constitutively active form of GOA-1, GOA-1(Q205L), inhibited axon regeneration ( Fig. 2a ; Supplementary Table S1 ). In addition, exogenous AEA did not enhance the regeneration defect in gain-of-function goa-1 mutants. These data suggest that the effect of AEA on regeneration is mediated by GOA-1. 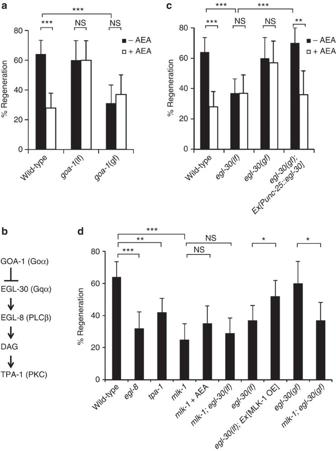Figure 2: Effects of GOA-1 and EGL-30 on axon regeneration. (a,c,d) Percentages of axons that initiated regeneration 24 h after laser surgery. Young adult animals were treated with ethanol (−AEA) or AEA for 6 h after axotomy. At least 30 axons in each condition were assayed. Error bars indicate 95% confidence interval (CI). *P<0.05, **P<0.01, ***P<0.001 as determined by Fisher's exact test. NS: not significant. (b) Schematic diagram showing the relationship between GOA-1 and EGL-30. Figure 2: Effects of GOA-1 and EGL-30 on axon regeneration. ( a,c,d ) Percentages of axons that initiated regeneration 24 h after laser surgery. Young adult animals were treated with ethanol (−AEA) or AEA for 6 h after axotomy. At least 30 axons in each condition were assayed. Error bars indicate 95% confidence interval (CI). * P <0.05, ** P <0.01, *** P <0.001 as determined by Fisher's exact test. NS: not significant. ( b ) Schematic diagram showing the relationship between GOA-1 and EGL-30. Full size image GOA-1 is known to antagonize the EGL-30 Gqα signalling cascade [22] , [23] ( Fig. 2b ). Hence, we hypothesised that EGL-30 would have an effect opposite to that of GOA-1 in axon regeneration. In fact, we found that loss-of-function egl-30(ad805) mutants exhibited a defect in axon regeneration ( Fig. 2c ; Supplementary Table S1 ). Moreover, a gain-of-function egl-30(tg26) mutation was able to suppress the defect in axon regeneration caused by the addition of AEA ( Fig. 2c ; Supplementary Table S1 ). When egl-30 was expressed in D-type motor neurons by the unc-25 promoter, the axon regeneration defect in egl-30(ad805) mutants was rescued and sensitivity to exogenous AEA was restored ( Fig. 2c ; Supplementary Table S1 ). Thus, EGL-30 functions cell autonomously in D-type motor neurons. Taken together, these results suggest that the AEA-GOA-1 signalling pathway inhibits axon regeneration by antagonizing EGL-30. One of the downstream effectors of EGL-30 is the phospholipase C β (PLCβ) homologue EGL-8 (24). PLCβ is known to generate diacylglycerol, which is a potent activator of protein kinase C (PKC) ( Fig. 2b ). Thus, we next asked if EGL-8 and PKC might control axon regeneration after laser surgery. We found that loss-of-function egl-8(nd971) mutants exhibited a defect in axon regeneration ( Fig. 2d ; Supplementary Table S1 ). C. elegans expresses the PKCδ isoform, TPA-1, which is activated by diacylglycerol [25] . The loss-of-function tpa-1(k501) mutation decreased the frequency of regeneration ( Fig. 2d ; Supplementary Table S1 ). These results suggest that TPA-1 functions as a downstream component of the EGL-30-EGL-8-stimulated signalling pathway that regulates axon regeneration after injury. Gqα and PKC function upstream of MLK-1 MAPKKK As our RNAi screen for svh genes was originally designed to identify regulators of the MAPK pathways [9] , we next investigated the relationship between AEA/EGL-30 and MAPK pathways in axon regeneration. The mlk-1(km19) null mutant lacks the MAPKKK that functions in the KGB-1 pathway [8] . In mlk-1(km19) mutants, about 25% of the axons were capable of regeneration ( Fig. 2d ; Supplementary Table S1 ) similar to the frequency observed in the presence of AEA or in loss-of-function egl-30 mutants. We therefore reasoned that AEA/EGL-30 might be involved in the MLK-1-MEK-1-KGB-1 JNK pathway. Consistent with this possibility, neither AEA treatment nor loss-of-function egl-30 mutation further inhibited axon regeneration in animals harbouring the mlk-1(km19) mutation ( Fig. 2d ; Supplementary Table S1 ). These results indicate that AEA/EGL-30 and MLK-1 act in the same pathway. We next examined the epistatic relationship between EGL-30 and MLK-1. Overexpression of mlk-1 partially suppressed the regeneration defect in egl-30(ad805) mutants ( Fig. 2d ) ( Supplementary Table S1 ). In contrast, the gain-of-function egl-30(tg26) mutation failed to suppress the mlk-1 defect ( Fig. 2d ; Supplementary Table S1 ). These results suggest that AEA/EGL-30 functions upstream of MLK-1 in axon regeneration. This genetic interaction between EGL-30 and MLK-1 raises the possibility that TPA-1 acts on MLK-1. To test this possibility, we examined the interaction between TPA-1 and MLK-1 by co-expressing T7-tagged TPA-1 and HA-tagged MLK-1 in COS-7 cells. We immunoprecipitated HA-MLK-1 with anti-HA antibody and probed for T7-TPA-1 on a western blot with anti-T7 antibody. We found that MLK-1 co-immunoprecipitated with TPA-1 ( Fig. 3a ), indicating that TPA-1 can physically associate with MLK-1. Next, we investigated whether TPA-1 phosphorylates MLK-1. MLK-1 contains a PKC phosphorylation consensus sequence (Arg-Xxx-Ser), which includes Ser-355 in the activation loop located between kinase subdomains VII and VIII ( Fig. 3b ). This phosphorylation is important for activation of MLK-1 kinase activity [26] , and this site is a likely target of TPA-1 kinase activity. We therefore asked whether TPA-1 phosphorylates MLK-1 at the Ser-355 residue. HA-MLK-1 was co-expressed with T7-TPA-1 in COS-7 cells, immunoprecipitated from cell lysates, and then analysed by western blotting with anti-phospho-MLK-1 antibody that specifically recognizes the phosphorylated Ser-355 form of MLK-1. Transfection with TPA-1 resulted in strong phosphorylation of MLK-1 ( Fig. 3b , lanes 1,2). Transfection with a catalytically inactive form of TPA-1(K404R) abrogated MLK-1 phosphorylation ( Fig. 3b , lane 4), indicating that the kinase activity of TPA-1 is required for phosphorylation of MLK-1. To confirm that TPA-1 phosphorylates MLK-1 Ser-355, we generated a mutant form of MLK-1 (MLK-1(S355A)), in which Ser-355 is mutated to alanine. When co-expressed with T7-TPA-1, MLK-1(S355A) was not detected by anti-phospho-MLK-1 antibody ( Fig. 3b , lane 3). 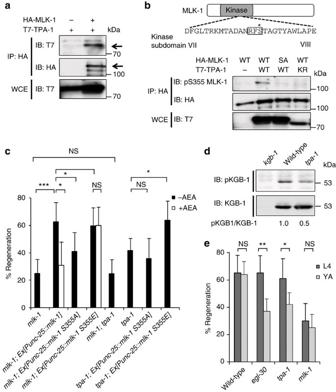Figure 3: The relationship between TPA-1 and MLK-1 in axon regeneration. (a) Interaction between TPA-1 and MLK-1. COS-7 cells were transfected with plasmids encoding T7-TPA-1 and HA-MLK-1 as indicated. Whole-cell extracts (WCE) and immunoprecipitated complexes obtained with anti-HA antibody (IP: HA) were analysed by immunoblotting (IB). Arrows indicate T7-TPA-1 and HA-MLK-1. (b) Phosphorylation of MLK-1 by TPA-1. Amino acid sequence of kinase subdomains VII and VIII in MLK-1 is shown in the upper part. The consensus site for PKC phosphorylation is boxed. The Ser-355 residue is indicated by an asterisk. COS-7 cells were transfected with plasmids encoding T7-TPA-1 (WT), T7-TPA-1(K404R) (KR), HA-MLK-1 (WT), and HA-MLK-1(S355A) (SA) as indicated. Whole-cell extracts and immunoprecipitated complexes obtained with anti-HA antibody were analysed by western blotting. pS355 MLK-1: anti-phospho-Ser-355 MLK-1 antibody. (c) Percentages of axons that initiated regeneration 24 h after laser surgery. Young adult animals were treated with ethanol (−AEA) or AEA for 6 h after axotomy. At least 30 axons in each condition were assayed. Error bars indicate 95% confidence interval (CI). *P<0.05, ***P<0.001 as determined by Fisher's exact test. NS, not significant. (d) Effect of thetpa-1mutation on KGB-1 activity. Extracts prepared from each animal were immunoblotted with anti-phospho-KGB-1 (pKGB-1) and anti-KGB-1 antibodies. pKGB-1 signal intensities were quantitated and normalized to the levels of KGB-1. Relative levels of pKGB-1 are shown. (e) Effect of age on axon regeneration. Animals in L4 or young adult (YA) stage were treated with ethanol for 6 h after axotomy. At least 30 axons in each condition were assayed. Error bars indicate 95% CI. *P<0.05, **P<0.01 as determined by Fisher's exact test. NS, not significant. Figure 3: The relationship between TPA-1 and MLK-1 in axon regeneration. ( a ) Interaction between TPA-1 and MLK-1. COS-7 cells were transfected with plasmids encoding T7-TPA-1 and HA-MLK-1 as indicated. Whole-cell extracts (WCE) and immunoprecipitated complexes obtained with anti-HA antibody (IP: HA) were analysed by immunoblotting (IB). Arrows indicate T7-TPA-1 and HA-MLK-1. ( b ) Phosphorylation of MLK-1 by TPA-1. Amino acid sequence of kinase subdomains VII and VIII in MLK-1 is shown in the upper part. The consensus site for PKC phosphorylation is boxed. The Ser-355 residue is indicated by an asterisk. COS-7 cells were transfected with plasmids encoding T7-TPA-1 (WT), T7-TPA-1(K404R) (KR), HA-MLK-1 (WT), and HA-MLK-1(S355A) (SA) as indicated. Whole-cell extracts and immunoprecipitated complexes obtained with anti-HA antibody were analysed by western blotting. pS355 MLK-1: anti-phospho-Ser-355 MLK-1 antibody. ( c ) Percentages of axons that initiated regeneration 24 h after laser surgery. Young adult animals were treated with ethanol (−AEA) or AEA for 6 h after axotomy. At least 30 axons in each condition were assayed. Error bars indicate 95% confidence interval (CI). * P <0.05, *** P <0.001 as determined by Fisher's exact test. NS, not significant. ( d ) Effect of the tpa-1 mutation on KGB-1 activity. Extracts prepared from each animal were immunoblotted with anti-phospho-KGB-1 (pKGB-1) and anti-KGB-1 antibodies. pKGB-1 signal intensities were quantitated and normalized to the levels of KGB-1. Relative levels of pKGB-1 are shown. ( e ) Effect of age on axon regeneration. Animals in L4 or young adult (YA) stage were treated with ethanol for 6 h after axotomy. At least 30 axons in each condition were assayed. Error bars indicate 95% CI. * P <0.05, ** P <0.01 as determined by Fisher's exact test. NS, not significant. Full size image To examine whether MLK-1 Ser-355 is functionally important in the regeneration pathway, wild-type MLK-1 and MLK-1(S355A) were expressed under the control of the unc-25 promoter in mlk-1(km19) null mutants. The Punc-25::mlk-1 fusion gene rescued the regeneration defect in mlk-1 mutants, whereas the MLK-1(S355A) mutated form did not ( Fig. 3c ; Supplementary Table S1 ). Furthermore, axon regeneration in mlk-1 mutants expressing wild-type MLK-1 could be inhibited by exogenous AEA ( Fig. 3c ; Supplementary Table S1 ). In contrast, expression of a phospho-mimetic form of MLK-1, MLK-1(S355E), in mlk-1(km19) mutants by the unc-25 promoter, conferred resistance to AEA-induced inhibition of axon regeneration ( Fig. 3c ; Supplementary Table S1 ). Thus, Ser-355 is important for MLK-1 function in the regulation of the regeneration pathway. Next we undertook a genetic approach to ask whether TPA-1 functions upstream of MLK-1 in axon regeneration. Animals harbouring both tpa-1 and mlk-1 mutations displayed regeneration frequency indistinguishable from that observed in the mlk-1 single mutants ( Fig. 3c ; Supplementary Table S1 ). This indicates that TPA-1 and MLK-1 are components of the same regeneration-promoting pathway. In addition, expression of MLK-1(S355E) was able to suppress the regeneration defect in tpa-1 mutants, whereas expression of MLK-1(S355A) was not ( Fig. 3c ; Supplementary Table S1 ). These results suggest that TPA-1 functions upstream of MLK-1 to promote axon regeneration. To confirm that TPA-1 functions in the MLK-1 pathway, we examined the effect of the tpa-1(k501) mutation on KGB-1 activation. MLK-1 phosphorylates and activates MEK-1, which in turn activates KGB-1 by phosphorylating it at the Ser-198 and Tyr-200 residues located between kinase subdomains VII and VIII [8] . Anti-phospho-KGB-1 (pKGB-1) antibody, which recognizes the phosphorylated form of KGB-1, was used to monitor KGB-1 activation in C. elegans [27] . Western blot analysis with anti-pKGB-1 antibody clearly detected the phosphorylated form of KGB-1 in wild-type animals, but not in kgb-1(km21) null mutants ( Fig. 3d ). We found that KGB-1 activity was decreased in tpa-1 mutants ( Fig. 3d ). Taken together, these results suggest that TPA-1 directly phosphorylates MLK-1 at the Ser-355 residue to activate MLK-1 kinase activity, resulting in activation of the KGB-1 pathway to promote axon regeneration. The above results suggest that AEA signalling regulates axon regeneration at the MLK-1 phosphorylation step. However, AEA treatment and the faah-1 mutation affected axon regeneration only when the lesion was made in young adult animals and not in L4 stage larvae ( Fig. 1e ; Supplementary Table S1 ). We next determined which step of the pathway is responsible for this developmental switch in regeneration ability. We found that egl-30(ad805) and tpa-1(k501) mutants were defective in axon regeneration as young adults but not at the L4 stage ( Fig. 3e ; Supplementary Table S1 ). In contrast, mlk-1(km19) null mutants were defective in regeneration at both the L4 larval and the young adult stages ( Fig. 3e ; Supplementary Table S1 ). These results suggest the existence of an AEA-insensitive mechanism of MLK-1 phosphorylation operating at the larval stage. The relationship between the SVH-1-SVH-2 and AEA pathways We have recently demonstrated that signalling mediated by the SVH-1 growth factor and SVH-2 tyrosine kinase receptor regulates axon regeneration through tyrosine phosphorylation of MLK-1 in the KGB-1 JNK pathway [9] ( Fig. 1a ). As AEA appears to influence regeneration through the same pathway, we examined the relationship between the SVH-1-SVH-2 and AEA pathways. The inhibition of regeneration observed in a svh-2(tm737) null mutant was not significantly affected by the addition of AEA ( Fig. 4a ; Supplementary Table S1 ). In addition, egl-30(ad805) or tpa-1(k501) mutations did not enhance the regeneration defect caused by the svh-2(tm737) mutation ( Fig. 4a ; Supplementary Table S1 ). These results suggest that the SVH-1-SVH-2 and AEA/EGL-30-TPA-1 pathways share the same downstream effector. 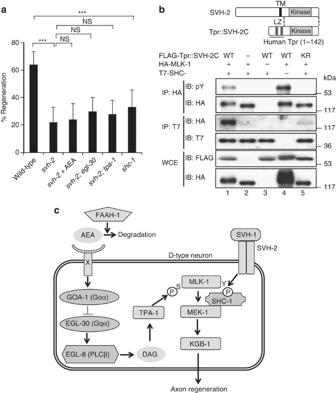Figure 4: Relationship between SVH-2 receptor tyrosine kinase and MLK-1 in axon regeneration. (a) Percentages of axons that initiated regeneration 24 h after laser surgery. Young adult animals were treated with ethanol or AEA for 6 h after axotomy. At least 30 axons in each condition were assayed. Error bars indicate 95% confidence interval (CI). ***P<0.001 as determined by Fisher's exact test. NS, not significant. (b) Effect of SVH-2 on the interaction between MLK-1 and SHC-1. Schematic diagrams of SVH-2 and Tpr::SVH-2C are shown in the upper part. COS-7 cells were transfected with plasmids encoding FLAG-Tpr::SVH-2C (WT), FLAG-Tpr::SVH-2C(K767R) (KR), HA-MLK-1 and T7-SHC-1 as indicated. Whole-cell extracts and immunoprecipitated complexes obtained with anti-HA (IP: HA) or anti-T7 antibody (IP: T7) were analysed by immunoblotting. pY: anti-phospho-tyrosine antibody. LZ: leucine zipper. (c) Schematic model for regulation of the KGB-1 JNK pathway by AEA-GOA-1/EGL-30-TPA-1 and SVH-1-SVH-2 in axon regeneration. Figure 4: Relationship between SVH-2 receptor tyrosine kinase and MLK-1 in axon regeneration. ( a ) Percentages of axons that initiated regeneration 24 h after laser surgery. Young adult animals were treated with ethanol or AEA for 6 h after axotomy. At least 30 axons in each condition were assayed. Error bars indicate 95% confidence interval (CI). *** P <0.001 as determined by Fisher's exact test. NS, not significant. ( b ) Effect of SVH-2 on the interaction between MLK-1 and SHC-1. Schematic diagrams of SVH-2 and Tpr::SVH-2C are shown in the upper part. COS-7 cells were transfected with plasmids encoding FLAG-Tpr::SVH-2C (WT), FLAG-Tpr::SVH-2C(K767R) (KR), HA-MLK-1 and T7-SHC-1 as indicated. Whole-cell extracts and immunoprecipitated complexes obtained with anti-HA (IP: HA) or anti-T7 antibody (IP: T7) were analysed by immunoblotting. pY: anti-phospho-tyrosine antibody. LZ: leucine zipper. ( c ) Schematic model for regulation of the KGB-1 JNK pathway by AEA-GOA-1/EGL-30-TPA-1 and SVH-1-SVH-2 in axon regeneration. Full size image The most likely candidate for this shared target is MLK-1. Therefore, we next asked how SVH-2 tyrosine kinase might regulate MLK-1 in this regeneration pathway. The C . elegans Shc adaptor protein SHC-1 is a crucial component of the KGB-1 pathway, and acts as a scaffold between MLK-1 and its immediate target MEK-1 MAPKK [27] . We found that 33% of shc-1(ok196) deletion mutants regenerated axons ( Fig. 4a ; Supplementary Table S1 ). This indicates that SHC-1 is indeed required for axon regeneration. As SHC-1 contains a phospho-tyrosine binding domain [27] , we tested the possibility that Tyr-phosphorylation of MLK-1 by SVH-2 creates a binding site for SHC-1. The tyrosine kinase activity of SVH-2 can be activated by fusing the N-terminus of a dimerization leucine zipper motif (Tpr: translocated promoter region) directly to the kinase domain and C-terminus of SVH-2 (9) ( Fig. 4b ). Consistent with this, immunoblot analysis with anti-phospho-tyrosine antibody (pY) revealed that co-expression of Tpr::SVH-2C induced tyrosine phosphorylation of MLK-1 ( Fig. 4b , first panel, lane 4). When HA-MLK-1 and T7-SHC-1 were co-expressed in mammalian COS-7 cells, immunoprecipitation analysis revealed that MLK-1 did not associate with SHC-1 ( Fig. 4b , third panel, lane 2). Co-expression of Tpr::SVH-2C with HA-MLK-1 and T7-SHC-1 induced tyrosine phosphorylation of MLK-1 ( Fig. 4b , first panel, lane 1) and association between MLK-1 and SHC-1 ( Fig. 4b , third panel, lane 1). However, a catalytically inactive mutant form, Tpr::SVH-2C(K767R), did not induce tyrosine phosphorylation of MLK-1 ( Fig. 4b , first panel, lane 5) and was unable to induce an association between MLK-1 and SHC-1 ( Fig. 4b , third panel, lane 5). These results suggest that the interaction between SHC-1 and MLK-1 depends on Tyr-phosphorylation of MLK-1 by SVH-2. C. elegans axon regeneration is regulated by the JNK MAPK pathway, which consists of MLK-1 (MAPKKK)-MEK-1 (MAPKK)-KGB-1 (JNK) [7] ( Fig. 4c ). We have recently demonstrated that the growth factor SVH-1 and its tyrosine kinase receptor SVH-2 promote axon regeneration through tyrosine phosphorylation of MLK-1 in the KGB-1 pathway [9] . The C . elegans Shc adaptor protein SHC-1 is an essential component of the KGB-1 pathway that acts as an adaptor to link MEK-1 MAPKK to MLK-1 MAPKKK [27] . In this study, we show that the interaction between SHC-1 and MLK-1 depends on SVH-2-mediated phosphorylation of the Tyr residue in MLK-1. Furthermore, we demonstrate that TPA-1 PKC phosphorylates the Ser residue in the activation loop of the MLK-1 kinase domain. Thus, MLK-1 is regulated by double phosphorylation ( Fig. 4c ), that is, TPA-1-mediated serine phosphorylation in the activation loop, which regulates its kinase activity, and SVH-2-mediated tyrosine phosphorylation, which regulates its association with SHC-1. As SHC-1 constitutively forms a complex with MEK-1, tyrosine phosphorylation of MLK-1 results in the recruitment of the SHC-1-MEK-1 complex to MLK-1. Loss-of-function mutations in egl-30 and tpa-1 cause defects in axon regeneration in young adult but not in L4 stage animals. By contrast, the mlk-1 null mutation affects axon regeneration at both the young adult and L4 stages. A possible explanation for this developmental switch is the existence of another protein kinase that functions redundantly with the EGL-30-TPA-1 pathway to mediate MLK-1 Ser phosphorylation in response to axon damage in larval-stage animals. Our findings reveal that AEA is a negative regulator of axon regeneration. This inhibitory effect is mediated by the Goα protein GOA-1, which antagonizes the EGL-30 Gqα-PKC-JNK cascade ( Fig. 4c ). These results indicate that axon regeneration of D-type motor neurons in wild-type animals is restrained by both extrinsic and intrinsic inhibitory factors. Thus, our results suggest a new role for AEA signalling in axonal regeneration. It will be interesting to determine whether endocannabinoids can affect axonal regeneration in mammals as well. In mammals, AEA is produced locally and transiently after several forms of injury, such as spinal cord injury and nerve inflammation [28] , [29] , protects nerve cells and enhances wound healing [30] , [31] . Therefore, it is possible that axon severing in C. elegans produces AEA around the damaged region, and that AEA transiently inhibits axon regeneration during the primary stage of healing. In mammals, the cannabinoid receptor is required for accurate growth cone steering of developing axons and subsequent synaptic connections in GABA-containing interneurons [15] , whereas its role in axon regeneration is unknown. Although C. elegans does not possess clear orthologues of the mammalian cannabinoid receptors [19] , we found that AEA regulates axon regeneration via Goα-dependent signalling. This suggests that there are unidentified G-protein coupled AEA receptors in C. elegans that are possibly conserved mediators of AEA signalling in axon regeneration. Identification of the functional cannabinoid receptor involved in mediating the inhibitory effect of AEA on regeneration would provide new avenues for research into the mechanisms of regeneration. This, in turn, would aid the development of therapeutic interventions to enhance regeneration or plasticity following nervous system injury. C. elegans strains The C. elegans strains used in this study are listed in Supplementary Table S2 . All strains were maintained on nematode growth medium plates and fed with bacteria of the OP50 strain [32] . The faah-1(tm5011) mutation is a deletion that includes the entire second exon, resulting in a frame shift with a stop codon appearing just after the transmembrane domain ( Supplementary Fig. S2 ). Chemicals AEA, EPEA, and 2-hydroxypropyl-β-cyclodextrin were obtained from Cayman Chemical, Fluorochem and Santa Cruz Biotechnology, respectively. Axotomy The regeneration ability of animals was assayed by a slightly modified version of a recently described regeneration assay [9] . Briefly, young adult or L4 hermaphrodite animals were immobilized with 20 mM levamisole solution in M9 buffer on a 2% agarose pad under a cover slip. D-type motor neurons expressing green fluorescent protein were imaged with a fluorescence microscope. Selected commissural axons, mainly posterior D-type neurons, were cut using a 440-nm MicroPoint ablation Laser System from Photonic Instruments. After surgery, animals were incubated for 6 h in M9 buffer solution containing 20 mM 2-hydroxypropyl-β-cyclodextrin [33] and either 2% ethanol (control), 290 μM AEA or 290 μM EPEA. Animals were transferred to an agar plate and remounted for fluorescent imaging ~24 h after surgery. Both Zeiss Axioplan fluorescent and Olympus FV-500 confocal laser microscopes were used for observation. Axons that grew a distance of 5 μm or more were scored as 'regenerated'. The proximal axon segments that showed no change after 24 h were counted as 'no regeneration'. At least 20 animals with 1–3 axotomized commissures were observed for most experiments. Two-tailed P -values were calculated using Fisher's exact test. Microscopy Standard fluorescent images of transgenic animals were observed under a Zeiss Plan-APOCHROMAT ×63 objective of a Zeiss Axioplan II fluorescent microscope and photographed with a Hamamatsu 3CCD camera. Confocal fluorescent images were taken on an Olympus FV-500 confocal laser-scanning microscope with a ×40 objective. RT–PCR Total RNA from faah-1(tm5011) mutants was extracted by the RNeasy kit (Qiagen) and reverse transcribed. The faah-1 cDNA was amplified by PCR with faah-1 specific primers: Forward primer: 5′-ACTTGGTGCTTCTCGTTTTGGG-3′. Reversed primer: 5′-GCTTCACGGAGTTCAAATGTGTC-3′. After this PCR amplification, the faah-1 cDNA was sequenced. Plasmids To make Pfaah-1::gfp , a 3-kb genomic DNA of the faah-1 promoter region in N2 was amplified by PCR with the following primers: F1: 5′-GCATGCgaatcttcatcctctgatggctgcat-3′; R1: 5′-GGTACCgatgaccttgaaatactgaaaattgaaagtg-3′. The primers introduced an Sph I (forward primer) and a Kpn I (reverse primer) endonuclease recognition sites. Using the SphI and KpnI sites, the amplified faah-1 promoter DNA was inserted into the pPD95.75 vector. Pmyo-2::faah-1 and Punc-25::faah-1 were generated by inserting the faah-1 cDNA isolated from a cDNA library [34] into the pPD30.69 vector and the pSC325 vector, respectively. Punc-25::egl-30, Punc-25::mlk-1 , Punc-25::mlk-1 (S355E) and Punc-25::mlk-1 (S355A) were generated by inserting egl-30 (yk343g12), mlk-1, mlk-1 (S355E) and mlk-1 (S355A) cDNAs [26] into the pSC325 vector. T7-TPA-1 was made by transferring TPA-1 cDNA [35] into a mammalian expression vector containing the cytomegalovirus promoter and encoding the T7 epitope [34] . T7-TPA-1(K404R) was made by oligonucleotide-directed PCR using T7-TPA-1 as a template and the mutation was verified by DNA sequencing. The primers used to introduce the K404R mutation are: F1: 5′-aatgagttttatgcaatgagatgtctgaaaaaggacgtg-3′; R1: 5′- cacgtcctttttcagacatctcattgcataaaactcatt-3′. Other plasmids, including FLAG-Tpr::SVH-2C, FLAG-Tpr::SVH-2C(K767R), T7-SHC-1 and Pmyo-2::dsredm , were previously described [9] , [27] , [36] . Transgenic animals Transgenic animals were obtained by a standard microinjection method of C. elegans [37] . Pmyo-2::faah-1 , Punc-25::faah-1 , Punc-25::egl-30 , a fosmid fragment containing the mlk-1 gene (as MLK-1 OE), Punc-25::mlk-1 , Punc-25::mlk-1 (S355A) and Punc-25::mlk-1 (S355E) (all 50 ng μl −1 ) plasmids were used in kmEx451 ( Pmyo-2::faah-1 + Pmyo-2::dsredm ), kmE457 ( Punc-25::faah-1 + Pmyo-2::dsredm ), kmEx452 ( Punc-25::egl-30 + Pmyo-2::dsredm ), kmEx453 (MLK-1 OE + Pmyo-2::dsredm ), kmEx454 ( Punc-25::mlk-1 + Pmyo-2::dsredm ), kmEx455 ( Punc-25::mlk-1 (S355A) + Pmyo-2::dsredm ) and kmE456 ( Punc-25::mlk-1 (S355E) + Pmyo-2::dsredm ), respectively. Biochemical analyses Transgenes were transfected into COS-7 cells by using FuGENE 6 transfection reagent (Roche) according to the manufacturer's instructions, and cells were harvested 48–72 h after transfection. Standard techniques were used for preparation of the cell lysates, immunoprecipitation and immunoblotting [34] . The worm extracts were prepared by boiling of harvested worms in SDS sample buffer. Anti-phospho-KGB-1, anti-KGB-1 and anti-phospho MLK-1 antibodies have been described previously [8] , [27] . We also used the following commercially available antibodies: anti-FLAG monoclonal antibody M2 (Sigma), anti-T7 monoclonal antibody (Novagen), anti-HA monoclonal antibody 16B12 (Covance), anti-phospho-tyrosine antibody PY20 (Upstate Inc.). Homology search and sequence alignment Homology search, detection of conserved domains and alignment of amino acids were executed by the NCBI BLAST and Genetyx-Mac programs. How to cite this article: Pastuhov, S. I. et al . Endocannabinoid-Goα signalling inhibits axon regeneration in Caenorhabditis elegans by antagonizing Gqα-PKC-JNK signalling. Nat. Commun. 3:1136 doi: 10.1038/ncomms2136 (2012).